Platelets promote tumour metastasis via interaction between TLR4 and tumour cell-released high-mobility group box1 protein Increasing evidence suggests that TLR4 expression by tumour cells promotes tumour progression, but it is unclear whether TLR4 is involved in metastasis. Here we show that TLR4 deficiency significantly diminishes experimental lung metastasis without affecting primary tumour growth. Bone marrow transplantation experiment and application of antiplatelet agents in mice demonstrate that TLR4 on platelets plays an important role in metastasis. TLR4 is critical for platelet–tumour cell interaction in vitro . Furthermore, high-mobility group box1 (HMGB1) neutralization attenuates platelet–tumour cell interaction in vitro and metastasis in vivo in a TLR4-dependent manner, indicating that tumour cell-released HMGB1 is the key factor that interacts with TLR4 on platelets and mediates platelet–tumour cell interaction, which promotes metastasis. These findings demonstrate a mechanism by which platelets promote tumour cell metastasis and suggest TLR4, and its endogenous ligand HMGB1 as targets for antimetastatic therapies. Metastasis constitutes the main cause of cancer-related death and a major challenge in today’s cancer management. Although many new therapies against malignant tumours have been developed over the past years, the prognosis of most malignancies remains unfavourable once metastatic spread has occurred. The metastatic process consists of a series of events: cell detachment from the primary tumour mass, migration into and transport along the bloodstream, and finally tumour cell arrest and proliferation within the distant tissue [1] . The mechanisms governing this clinically important process remain poorly understood. Metastasis is a highly inefficient process, as <0.1% of tumour cells that penetrate the circulation end up forming metastatic colonies [2] , [3] . Most of the tumour cells introduced into the circulation are rapidly eliminated by shear stress or immune cells [4] . There is a plethora of studies indicating that the interaction of tumour cells with platelets within the bloodstream is essential during this early phase of metastasis [5] , [6] , [7] , and the ability of the circulating tumour cells to interact with platelets promote their survival within the circulation and therefore facilitate metastasis [4] , [5] . Platelets are involved in formation of a thrombus around tumour cells within the bloodstream, thus protecting tumour cells from shear stresses and natural killer (NK) cells lysis [8] . Coating circulating cancer cells with platelets enhances their extravasation by increasing their adhesion to the vessel wall [9] . Platelets can release multiple cytokines and chemokines participating in the tumour cell extravasation, angiogenesis and vascular remodelling [5] . Platelet-specific proteins such as P-selectin and αIIbβ3 mediate interactions among tumour cells, platelets, fibrin and so on to form an embolus [10] . Moreover, the platelets–tumour cell interaction can lead to the transfer of the platelet major histocompatibility complex-I to tumour cells, thereby preventing NK cell recognition [11] and the epithelial–mesenchymal-like transition (EMT) of tumour cells through the transforming growth factor-β (TGFβ) and nuclear factor-κB pathway, thus promoting metastasis [12] . Studies using transgenic mice models deficient in key platelet molecules (such as NFE2, PAR4 and P-selectin) further refine the notion that platelets have crucial roles in tumour metastasis [5] . Toll-like receptor 4 (TLR4) has been implicated in both microbial and sterile inflammation by responding to both bacterial endotoxin and multiple endogenous ligands [13] . Depending on the composition of the cells in the microenvironment and stage of disease, activation of TLR4 signalling can either stimulate [14] or inhibit [15] tumour development. Studies focusing on the endotoxin and tumour cell TLR4 have already shown that endotoxin is a potent promoter of tumour metastasis when infused systemically [16] , and that tumour cell TLR4 activation by endotoxin resulted in EMT of tumour cells and augmented metastasis [17] . Importantly, TLR4 can detect endogenous damage-associated molecular patterns including the widely expressed alarmin protein HMGB1 (ref. 18 ). HMGB1 is a nuclear constituent loosely bound to chromatin. When it is released from necrotic cells or secreted by activated macrophages, it acts like a cytokine involved in inflammation and tumour progression [18] . It is reported that the action of HMGB1, which is released by dying tumour cells, on TLR4 expressed by dendritic cells led to the activation of tumour antigen-specific T-cell immunity, resulting in tumour suppression [15] . However, whether host TLR4 is involved in tumour metastasis is unclear. Platelets express all the components of the lipopolysaccharide (LPS) receptor signalling complex (including TLR4, CD14, MD2 and myeloid differentiation primary response protein 88) [19] , [20] , [21] . During sepsis, TLR4 expressed on platelets serves as a bridge between platelets and other immune cells [22] . The recognition of pathogen molecules by TLR4 on platelets is linked to activation of innate immune system and contribute to pathogen recognition and to the inhibition of pathogen spreading in vivo [22] . In addition, TLR4 on platelets is the determining factor of LPS-induced thrombocytopenia and platelet aggregation in the lung and liver microvascular circulation in mice [23] . In vitro studies showed that platelet binds to fibrinogen under flow conditions in a TLR4-dependent manner [19] ; LPS stimulates platelet secretion and potentiates platelet aggregation through a TLR4/MyD88-dependent pathway [21] . In spite of the roles of the platelet TLR4 in immune regulation, the role of the platelet TLR4 in tumour progression and metastasis has not been directly characterized. The crucial roles of platelets in tumour metastasis, the involvement of TLR4 in tumour promotion and the relative high levels of TLR4 in platelets prompted us to investigate whether TLR4 is involved in tumour metastasis and whether TLR4 affects platelet function in this process, using in vivo and in vitro models. Here we show that platelets promote experimental tumour metastasis of murine B16F10 melanoma and Lewis lung carcinoma (LLC) tumour cells via interaction between platelet TLR4 and tumour cell-released HMGB1. Our findings demonstrate that TLR4 is an attractive target against platelet-mediated enhancement of tumour metastasis and that targeting TLR4 or its endogenous ligand HMGB1 is a novel therapeutic strategy for combating life-threatening metastasis. Experimental metastasis is diminished in TLR4-deficient mice To directly test the hypothesis that TLR4 signalling has a role in tumour metastasis, we used two well-studied mouse models [24] . The increasing numbers of B16F10 melanoma cells or LLC cells were injected into the tail vein of the wild-type (WT) and TLR4 −/− mice, and the extent of lung metastasis was determined later. Both B16F10 and LLC cells were capable of establishing pulmonary metastatic foci in mice; however, the formation of pulmonary metastatic foci was significantly decreased in TLR4 −/− mice compared with WT mice ( Fig. 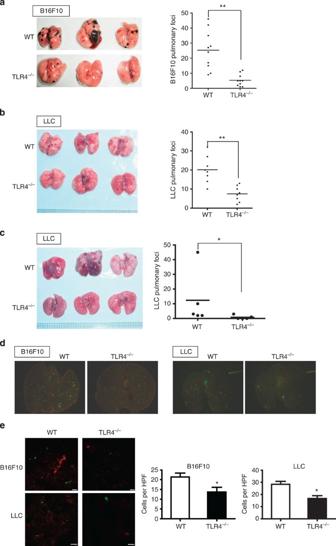Figure 1: Host TLR4 deficiency diminish tumour metastasis. (a,b) Representative photographs of pulmonary metastatic foci produced 14 days after i.v. injection of B16F10 cells (a,n=10 per group) or 21 days after i.v. injection of LLC cells (b,n=7 or 8 per group). The numbers of lung metastases are shown in the right (Mann–WhitneyU-test; **P<0.01). (c) Representative photograph of metastatic LLC foci in the lung from WT andTLR4−/−mice. The numbers of lung metastases are shown in the right (Mann–WhitneyU-test; *P<0.05;n=5 per group). (d) Fluorescence stereomicroscopy of lungs at 6 h after tail vein injection of 1 × 106CFSE-labelled B16F10 or LLC cells isolated from WT andTLR4−/−mice. Exposure time was constant. Three mice per group were studied. (e) Tumour cell engrafted in the lungs were determined using fluorescent microscopy. Green, CFSE-labelled B16F10 or LLC cells; red, DyLight 594-L. esculentum(Tomato) lectin. Scale bar, 50 μm. The numbers of cells engrafted in the lung per high power field (HPF; × 200) are shown in the right panel. Three mice were analysed in each group of this study. Data are presented as mean±s.e.m. *P<0.05, Student’st-test. Data are representative of three independent experiments. 1a,b and Table 1 ). To rule out the possibility that TLR4 may affect tumour growth, the size distribution of lung metastatic foci were determined. There was no obvious difference in the size or distribution of the metastatic foci that formed in control and TLR4-deficient mice ( Supplementary Tables 1 and 2 ). In agreement with these findings, the growth rate of primary tumours formed by subcutaneously injected B16F10 and LLC cells showed no difference between WT and TLR4 −/− mice over a 14-day observation period ( Supplementary Fig. 1 ). Spontaneous transplant models of metastasis encompass early and late stages of metastasis, and involve the transplantation of cells into either an ectopic or orthotopic site to form a primary tumour, which may subsequently metastasize [24] , [25] . We then determined the effects of host TLR4 deficiency on spontaneous metastasis using LLC cells by injection of the cells subcutaneously. As shown in Fig. 1c , the metastatic tumour number was significantly lower in TLR4 −/− mice than in WT mice. Moreover, all the WT mice (five out of five) developed apparent metastatic foci in the lung, whereas only two out of five TLR4 −/− mice developed metastasis. Figure 1: Host TLR4 deficiency diminish tumour metastasis. ( a , b ) Representative photographs of pulmonary metastatic foci produced 14 days after i.v. injection of B16F10 cells (a, n =10 per group) or 21 days after i.v. injection of LLC cells (b, n =7 or 8 per group). The numbers of lung metastases are shown in the right (Mann–Whitney U -test; ** P <0.01). ( c ) Representative photograph of metastatic LLC foci in the lung from WT and TLR4 −/− mice. The numbers of lung metastases are shown in the right (Mann–Whitney U -test; * P <0.05; n =5 per group). ( d ) Fluorescence stereomicroscopy of lungs at 6 h after tail vein injection of 1 × 10 6 CFSE-labelled B16F10 or LLC cells isolated from WT and TLR4 −/− mice. Exposure time was constant. Three mice per group were studied. ( e ) Tumour cell engrafted in the lungs were determined using fluorescent microscopy. Green, CFSE-labelled B16F10 or LLC cells; red, DyLight 594- L. esculentum (Tomato) lectin. Scale bar, 50 μm. The numbers of cells engrafted in the lung per high power field (HPF; × 200) are shown in the right panel. Three mice were analysed in each group of this study. Data are presented as mean±s.e.m. * P <0.05, Student’s t -test. Data are representative of three independent experiments. Full size image Table 1 Effect of host TLR4 deficiency on tumour metastasis. Full size table Distant metastases rely on haematogenous dissemination via the blood circulation, and the initial hours after tumour cell entering into circulation are crucial for successful metastasis [4] . To gain insight into why metastases were diminished in TLR4 −/− mice, WT and TLR4 −/− mice were administered with equal number of 5-(and-6)-carboxyfluorescein diacetate, succinimidyl ester (CFSE)-labelled B16F10 cells intravenously (i.v. ), and 6 h later the tumour cell distribution was analysed using stereo microscope. As shown in Fig. 1d , there was an apparent decrease in the tumour load in TLR4 −/− lungs compared with WT lungs. Immunofluorescence analysis revealed that CFSE-labelled tumour cells were mainly localized away from Lectin-positive vasculature ( Fig. 1e ) at this time point, indicating the extravasation of the engrafted tumour cells. In accordance, significantly more tumour cells could be observed in WT lungs than in TLR4 −/− lungs. These data suggest that host TLR4 deficiency reduced the lung retention and engraftment of the infused tumour cells. Host TLR4 activation promotes metastasis It is well documented that LPS, the ligand of TLR4, had potent facilitating effect on experimental metastasis when administrated intraperitoneally (i.p.) [16] and LPS-pretreated cells had increased metastatic potential [26] . To further verify that host TLR4 activation promoted metastasis, we determined the effects of LPS (to activate TLR4) or TLR4 antagonist on metastasis. WT and TLR4 −/− mice were administered with LPS 6 h before tumour cell injection and the tumour load in the lungs were determined 14 days later. Although LPS promoted lung metastasis in both genotypes, TLR4 −/− mice had much fewer lung metastatic foci compared with the similarly treated WT mice, indicating that host TLR4 activation potently promotes tumour metastasis ( Fig. 2a ). Next, we determined the effect of TLR4 blockage on tumour metastasis. TAK-242, a cyclohexene derivative, is a novel small-molecule compound that selectively inhibits TLR4 signalling [27] and has been shown effective in protecting mice against LPS-induced lethality [28] . Mice were administered with TAK-242, followed by tumour cell injection 1 h later. As expected, the TAK-242 inhibited tumour metastasis in WT mice, but had little effect in TLR4-deficient mice ( Fig. 2b ). Collectively, these data confirmed that host TLR4 activation promotes tumour metastasis. 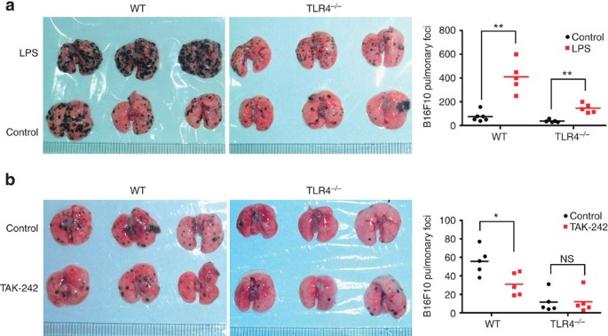Figure 2: Host TLR4 activation promotes tumour metastasis. (a) WT andTLR4−/−mice were injected with LPS i.p., followed by B16F10 infusion i.v. 6 h later. Fourteen days later, the lungs were isolated and representative photographs are shown. The number of metastatic foci is shown in the right panel (n=5 per group). (b) WT andTLR4−/−mice were injected with TAK-242 i.p., followed by B16F10 infusion i.v. 1 h later. Fourteen days later, the lungs were isolated and representative photographs were shown. The number of metastatic foci was shown in the right panel (n=5 per group). *P<0.05; **P<0.01; calculated by Mann–WhitneyU-test. Data are representative of three independent experiments. Figure 2: Host TLR4 activation promotes tumour metastasis. ( a ) WT and TLR4 − / − mice were injected with LPS i.p., followed by B16F10 infusion i.v. 6 h later. Fourteen days later, the lungs were isolated and representative photographs are shown. The number of metastatic foci is shown in the right panel ( n =5 per group). ( b ) WT and TLR4 −/− mice were injected with TAK-242 i.p., followed by B16F10 infusion i.v. 1 h later. Fourteen days later, the lungs were isolated and representative photographs were shown. The number of metastatic foci was shown in the right panel ( n =5 per group). * P <0.05; ** P <0.01; calculated by Mann–Whitney U -test. Data are representative of three independent experiments. Full size image TLR4 on haematopoietic-derived cells promotes metastasis To investigate whether the diminution in metastasis observed in TLR4 −/− mice was due to the absence of TLR4 within cells of haematopoietic origin, we limited the genetic deficit in TLR4 to haematopoietic-derived cells by bone marrow transplantation (BMT). Similar to the findings in the straight TLR4 knockout, mice that received transplants of bone marrow from TLR4-deficient donors developed far fewer pulmonary and liver metastases than mice that received transplants of bone marrow from WT donors ( Fig. 3a,b ). 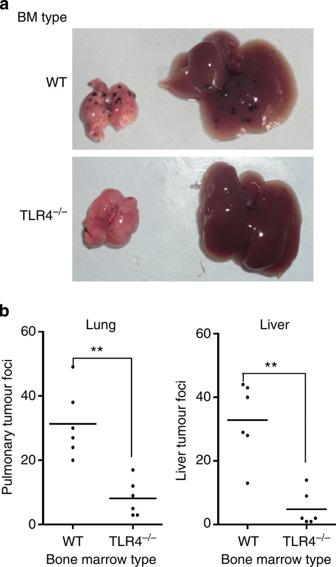Figure 3: TLR4 expressed on myeloid cells facilitates tumour metastasis. (a,b) Irradiated WT mice were reconstituted with WT orTLR4−/−bone marrow and then injected with B16F10 cells i.v. Fourteen days later, the lung and liver metastases were determined (a). The numbers of lung and liver metastatic foci are shown inb; (Mann–WhitneyU-test. *P<0.05; **P<0.01;n=6 per group). Data are representative of three independent experiments. Figure 3: TLR4 expressed on myeloid cells facilitates tumour metastasis. ( a , b ) Irradiated WT mice were reconstituted with WT or TLR4 −/− bone marrow and then injected with B16F10 cells i.v. Fourteen days later, the lung and liver metastases were determined ( a ). The numbers of lung and liver metastatic foci are shown in b ; (Mann–Whitney U -test. * P <0.05; ** P <0.01; n =6 per group). Data are representative of three independent experiments. Full size image To explore in greater detail which type of haematopoietic cells play a part in the tumour metastasis, we first performed routine blood tests in WT and TLR4 −/− mice. As shown in Fig. 4a , there was no significant difference in the amount of red blood cells, haemoglobin and white blood cells between WT and TLR4 −/− mice. However, total number of circulating platelets was slightly lower in TLR4 −/− mice than in WT mice, which was consistent with the previous reports [29] , [30] . Notably, when mice were administered with a bolus injection of B16F10 cells, significant thrombocytopenia appeared in WT but not in TLR4 −/− mice ( Fig. 4b ). Given the important roles of platelets in tumour metastasis, especially in the initial hours of this process [4] , [5] , we wondered whether TLR4 deficit affects the functions of platelets in tumour metastasis. The activation state of platelets was determined in tumour-bearing mice by analysing the expression of P-selectin on platelets using flow cytometry. As shown in Fig. 4c , compared with WT mice, the expression of P-selectin on TLR4 −/− platelets was much lower, indicating the attenuated activation of platelets. In accordance, the plasma levels of soluble P-selectin were consistently lower in TLR4 −/− than in WT mice ( Supplementary Fig. 2a ). Furthermore, the levels of TGFβ1, a platelet-derived cytokine involved in tumour metastasis [12] , [31] , [32] , were also significantly decreased in TLR4 −/− mice ( Fig. 4d and Supplementary Fig. 2b ). In addition, the plasma level of TXA2, a product of activated platelets and a potent agonist of platelet activity [33] , was significantly lower in tumour-bearing TLR4 −/− mice than that in WT mice ( Supplementary Fig. 2c ). These data suggest that TLR4 deficiency led to decreased platelet activation on tumour cell infusion. 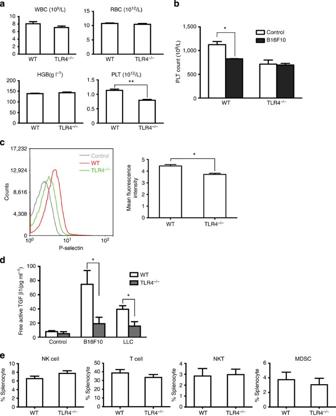Figure 4:TLR4deficiency inhibits tumour-induced platelet activation. (a) Blood routine tests were performed in WT andTLR4−/−mice (n=6 per group). (b) WT andTLR4−/−mice were injected with 1 × 106B16F10 cells i.v., and 30 min later the platelet numbers were determined (n=5 per group). (c) WT andTLR4−/−mice were injected with B16F10 cells i.v. Fourteen days later, expression of P-selectin on platelets was analysed by flow cytometry. Quantitative results are expressed as mean fluorescence intensity of P-selectin (n=5 per group). (d) The levels of free active TGFβ1 in the plasma of tumour-bearing mice were determined by ELISA (n=5 per group). (e) The percentage of NK, T, NKT and MDSC cells in the spleen was determined with flow cytometry (n=5 per group). Data are presented as mean±s.e.m. *P<0.05; **P<0.01; Studentt-test. All the experiments were replicated at least three times. Figure 4: TLR4 deficiency inhibits tumour-induced platelet activation. ( a ) Blood routine tests were performed in WT and TLR4 −/− mice ( n =6 per group). ( b ) WT and TLR4 −/− mice were injected with 1 × 10 6 B16F10 cells i.v., and 30 min later the platelet numbers were determined ( n =5 per group). ( c ) WT and TLR4 −/− mice were injected with B16F10 cells i.v. Fourteen days later, expression of P-selectin on platelets was analysed by flow cytometry. Quantitative results are expressed as mean fluorescence intensity of P-selectin ( n =5 per group). ( d ) The levels of free active TGFβ1 in the plasma of tumour-bearing mice were determined by ELISA ( n =5 per group). ( e ) The percentage of NK, T, NKT and MDSC cells in the spleen was determined with flow cytometry ( n =5 per group). Data are presented as mean±s.e.m. * P <0.05; ** P <0.01; Student t -test. All the experiments were replicated at least three times. Full size image Recruitment of immune cells, such as T cells, NK cells, NKT cells and myeloid-derived suppressor cells (MDSCs) can affect the tumour burden in the lung [34] , [35] , [36] , [37] . Therefore, we determined the changes in the composition of immune cell subsets of splenocytes, blood and metastatic tumour foci in the lung in tumour-bearing mice. As shown in Fig. 4e and Supplementary Fig. 3a,b , relative immune cell percentages from the spleen, blood and metastatic foci in the lung were not significantly different between WT and TLR4 −/− mice. Based on these data, we postulated that the reduced metastasis seen in TLR4 −/− mice is due to TLR4 deficiency in platelets. TLR4 on platelets promotes metastasis To illustrate whether TLR4 deficiency in platelets inhibits metastasis, we determined the direct effects of platelets on tumour cells. B16F10 cells were co-cultured with platelets from WT or TLR4-deficient mice for 40 h and then injected into WT or TLR4 −/− mice. Experimental metastasis analysis showed that despite the significant difference of metastasis between WT and TLR4 −/− recipient mice, pretreatment with WT but not TLR4 -null platelets led to increased B16F10 cell metastatic potential in both types of recipient mice ( Fig. 5a ). These data further confirmed the requirement of host TLR4 for efficient metastasis. Importantly, a platelet pretreatment primes tumour cells for metastasis in a TLR4-dependent manner, suggesting that TLR4 is involved in platelet–tumour cell interaction, which is of great importance in metastasis. 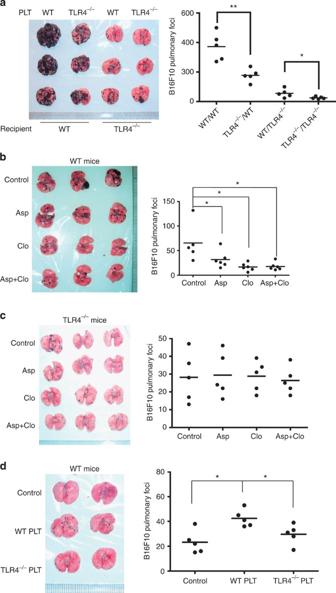Figure 5: Anti-platelet drugs inhibit metastasis in WT but not inTLR4−/−mice. (a) B16F10 cells were pretreated with WT orTLR4−/−platelets for 24 h and then injected into WT orTLR4−/−mice i.v. The lung metastases were determined 14 days later. WT mice (b) orTLR4−/−mice (c) injected with B16F10 cells i.v. were treated with Aspirin (Asp), Clopidogrel (Clo) or Asp+Clo in drinking water. Fourteen days later, lung metastases were determined. (d) WT mice were infused with WT,TLR4−/−platelets or buffer (Control) and B16F10 cells i.v. and the lung metastases were determined 14 days later.n=5 per group. *P<0.05; **P<0.01.P-value was calculated by Mann–WhitneyU-test. Data are representative of three independent experiments. Figure 5: Anti-platelet drugs inhibit metastasis in WT but not in TLR4 −/− mice. ( a ) B16F10 cells were pretreated with WT or TLR4 −/− platelets for 24 h and then injected into WT or TLR4 −/− mice i.v. The lung metastases were determined 14 days later. WT mice ( b ) or TLR4 −/− mice ( c ) injected with B16F10 cells i.v. were treated with Aspirin (Asp), Clopidogrel (Clo) or Asp+Clo in drinking water. Fourteen days later, lung metastases were determined. ( d ) WT mice were infused with WT, TLR4 −/− platelets or buffer (Control) and B16F10 cells i.v. and the lung metastases were determined 14 days later. n =5 per group. * P <0.05; ** P <0.01. P -value was calculated by Mann–Whitney U -test. Data are representative of three independent experiments. Full size image Considering the fact that platelets primarily act at the early time of metastasis [4] , [5] , it is important to elucidate the role of platelet TLR4 in metastasis in vivo . Tumour cells can induce platelet activation through various mechanisms and their metastatic potential correlates with their ability to activate platelets [37] , [38] , [39] , [40] . Pharmacological inhibition of platelet activation [41] , or depletion [5] or inhibition [42] of proteins critical for platelet activation significantly decreased the metastatic potential of tumour cells. To test whether the metastasis-enhancing effect of platelet was dependent on TLR4, WT and TLR4 −/− mice were treated with two mechanistically different antiplatelet agents. Aspirin causes irreversible inhibition of cyclooxygenase-1 in platelets and subsequent TXA2 production, while clopidogrel antagonizes the P2Y12 ADP receptor [43] . In WT mice both of them significantly inhibited metastasis ( Fig. 5b ), whereas in TLR4-deficient mice none of them was able to reduce lung metastasis ( Fig. 5c ). Moreover, there was no significant difference in the size distribution of metastatic foci formed in WT mice treated with or without antiplatelet agents, suggesting that antiplatelet agents did not affect tumour growth ( Supplementary Table 3 ). As these two drugs inhibited platelet activation (indicated by the levels of TXB2, Supplementary Fig. 2d ) but did not reduce the number of platelets [44] , these data also suggest that TLR4 deficiency in platelets may inhibit tumour cell-induced platelet activation. We next tested whether platelet infusion could promote tumour metastasis. WT mice were injected with B16F10 cells by tail vein, and on the opposite tail vein, with 1 × 10 9 platelets isolated from WT mice or TLR4 −/− mice. The platelets were infused every 5 days. Fourteen days later, the mice were killed and the lungs were isolated. As shown in Fig. 5d , mice administrated with WT platelets developed more tumour nodules in their lungs than mice administrated with buffer or TLR4 −/− platelets. Collectively, these data show that TLR4 on platelets has potent facilitating effects on tumour metastasis. Moreover, these data also show that TLR4 on platelets is involved in tumour cell-induced platelet activation. TLR4 deficiency impairs platelet–tumour cell interaction The in vivo results that inhibition of platelet activation reduces metastasis while reconstitution of WT platelets restores metastatic activity prompted us to investigate the role of TLR4 in platelet–tumour cell interaction. First, adhesion of platelets to tumour cells under static conditions was determined based on the fluorescent detection of CFSE-labelled platelets. Tumour cells were co-cultured with CFSE-labelled platelets for the indicated times. After the non-adherent platelets were washed away, the remaining fluorescence around the tumour cells was determined using a spectrophotometer and the platelet adhesion rate was calculated. As shown in Fig. 6a , the WT platelets were more prone to adhesion to tumour cells than TLR4 −/− platelets. The cell cultures were also analysed using a confocal microscope. As shown in Fig. 6b , the WT platelets formed the rosette-like structure around the tumour cells; however, this structure was rare in the TLR4 −/− platelet-treated tumour cells. We also determined the adhesion of platelets to tumour cells in vivo . CFSE-labelled platelets and PKH-26-labelled B16F10 cells were injected into antibody-induced thrombocytopenia mice via opposite tail veins; 6 h later, the lungs were isolated, cryosectioned and examined using fluorescent microscope. As shown in Fig. 6c , the number of tumour cells surrounded with platelets was much more in the WT platelet-infused mice than in mice infused with TLR4 −/− platelets. These results suggest the involvement of TLR4 in the interaction of platelets with tumour cells. 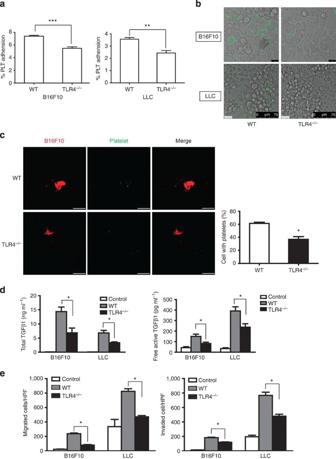Figure 6: TLR4-null platelets are impaired in tumour cell interaction. (a) Platelet adhesion to B16F10 or LLC cells was quantified based on the fluorescence detection of CFSE-labelled platelets as described in ‘Methods’. (b) Fluorescence microscopy images of CFSE-labelled platelets adhering to B16F10 and LLC cells. Noting the rosette-like structures in the WT platelets-group. Scale bar, 25 μm (upper panels) or 75 μm. (c) Mice were injected i.v. with 100 μg anti-CD41 antibody 3 h before CFSE-labelled platelets (green) and PKH26-labelled B16F10 (red) cells injection. After 6 h, the lungs were isolated and the co-localization of B16F10 cells with platelets was determined using a fluorescent microscopy. The numbers of tumour cells co-localized with platelets are shown in the right. Three mice per group were studied. Scale bar, 10 μm. (d) Tumour cells were co-cultured with WT orTLR4−/−platelet for 24 h. The levels of total and free active TGFβ1 in the mediums were determined by ELISA (Student’st-test). (e) B16F10 and LLC cells were seeded in Transwell inserts (left panel) or Matrigel invasion chambers (right panel), and treated with WT orTLR4−/−platelets. Twenty-four or 36 h later, the migrated cells were counted. Data are representative of three independent experiments. Data are presented as mean±s.e.m. *P<0.05; **P<0.01; ***P<0.001; calculated by Studentt-test. Figure 6: TLR4-null platelets are impaired in tumour cell interaction. ( a ) Platelet adhesion to B16F10 or LLC cells was quantified based on the fluorescence detection of CFSE-labelled platelets as described in ‘Methods’. ( b ) Fluorescence microscopy images of CFSE-labelled platelets adhering to B16F10 and LLC cells. Noting the rosette-like structures in the WT platelets-group. Scale bar, 25 μm (upper panels) or 75 μm. ( c ) Mice were injected i.v. with 100 μg anti-CD41 antibody 3 h before CFSE-labelled platelets (green) and PKH26-labelled B16F10 (red) cells injection. After 6 h, the lungs were isolated and the co-localization of B16F10 cells with platelets was determined using a fluorescent microscopy. The numbers of tumour cells co-localized with platelets are shown in the right. Three mice per group were studied. Scale bar, 10 μm. ( d ) Tumour cells were co-cultured with WT or TLR4 −/− platelet for 24 h. The levels of total and free active TGFβ1 in the mediums were determined by ELISA (Student’s t -test). ( e ) B16F10 and LLC cells were seeded in Transwell inserts (left panel) or Matrigel invasion chambers (right panel), and treated with WT or TLR4 −/− platelets. Twenty-four or 36 h later, the migrated cells were counted. Data are representative of three independent experiments. Data are presented as mean±s.e.m. * P <0.05; ** P <0.01; *** P <0.001; calculated by Student t -test. Full size image Platelets can promote tumour metastasis by releasing a plethora of bioactive factors including TGFβ1, which is crucial for metastasis [12] (see Fig. 4d and Supplementary Fig. 2b ). We then analysed TGFβ1 secretion from platelets on exposure to tumour cells in vitro . When co-cultured with tumour cells, the WT platelets released more TGFβ1 than TLR4 −/− platelets did ( Fig. 6d ). Next, we tested the metastasis-promoting effects of platelets in vitro using the migration assay and invasion assay. B16F10 and LLC cells were mixed with WT, TLR4 −/− platelets or buffer control and seeded on transwell inserts or Matrigel-coated inserts; 24 h later, the migrated cells were counted. Platelets treatment significantly enhanced tumour cell migration and invasion, whereas inhibition of TGFβ signalling reduced such effects ( Supplementary Fig. 4a,b ). Compared with WT platelet-treated group, TLR4 −/− platelet-treated tumour cells showed significantly attenuated migration and invasiveness ( Fig. 6e and Supplementary Fig. 5a,b ). To investigate whether platelet–tumour cell contact is necessary for the metastasis-promoting effects, tumour cells were seeded on the Matrigel-coated inserts, while WT or TLR4 −/− platelets were seeded on the bottom chamber to avoid their direct contact and cultured for 24 h at 37 °C. No significant difference was observed between two wells ( Supplementary Fig. 5c ), suggesting that platelet–tumour cell contact is necessary for TLR4-dependent metastasis-promoting effects of platelets. HMGB1 mediates platelet–tumour cell interaction Next, we sought to find out the factor that mediates platelet–tumour cell interaction. The tumour metastasis is a relatively ineffective process, as most cells are destroyed in the blood due to sheer stress or lysis by NK cells [8] . The destroyed tumour cells can release factors to stimulate the host cells [45] . The alarmin protein HMGB1, an endogenous ligand of TLR4, is one of the key factors released by necrotic cells, playing critical roles at the intersection of the host inflammatory response to sterile and infectious threat [18] , [46] . It is released by injured cells in the absence of exogenous agents or by cells exposed to pathogen-derived molecules, and its binding and signalling through TLR4 mediate cytokine release and tissue injury in animal models of infection, ischaemia and injury [18] . When tumour cells were injected either i.v. or subcutaneously, the levels of HMGB1 were elevated to a much higher extent in the circulation of WT mice than TLR4 −/− mice ( Fig. 7a,b ). Importantly, HMGB1 was present in microvesicles, indicative of active release from B16F10 and LLC ( Supplementary Fig. 6a ). To determine whether HMGB1 is involved in platelet–tumour cell interaction, a HMGB1 neutralizing antibody was used [47] . When tumour cells were co-cultured with WT platelets, HMGB1 neutralization led to the reduced adhesion of platelets to tumour cells ( Fig. 7c ). Furthermore, TGFβ1 release from tumour cell-treated platelets was dramatically reduced, indicating a critical role of tumour cell-derived HMGB1 in TGFβ1 release ( Fig. 7d ). In addition, invasion assay showed that anti-HMGB1 antibody treatment significantly attenuated platelet-induced tumour cell invasion ( Fig. 7e and Supplementary Fig. 6b,c ). However, all these effects of HMGB1 neutralization were only seen in WT platelets but not in TLR4 −/− platelets. We also determined the effects of anti-HMGB1 antibody on metastasis in vivo . Both WT and TLR4 −/− mice were injected with B16F10 cells and treated with anti-HMGB1 antibody. Fourteen days later, the lung metastasis was assessed. As shown in Fig. 7f , HMGB1 neutralization significantly reduced experimental metastasis in WT mice but not in TLR4 −/− mice, suggesting that HMGB1 signals through TLR4 to promote metastasis. 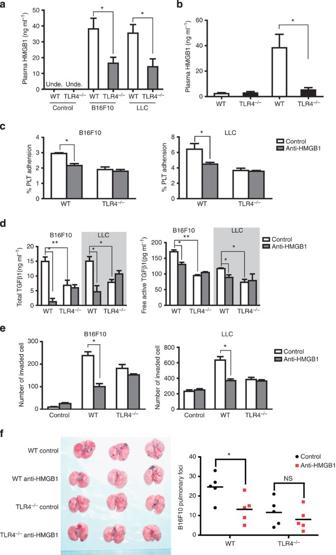Figure 7: HMGB1 plays a crucial role in platelet–tumour cell interaction. (a) The levels of HMGB1 in the plasma of tumour-bearing mice were detected by ELISA. (Student’st-test;n=5 per group). (b) The levels of HMGB1 in the plasma of mice with spontaneous LLC metastases were detected by ELISA. (Student’st-test;n=5 per group). (c) Platelet adhesion to B16F10 or LLC cells with or without 5 μg ml−1anti-HMGB1 was quantified based on the fluorescence detection of CFSE-labelled platelets as described in ‘Methods’ (Student’st-test). (d) B16F10 or LLC cells were co-cultured with WT orTLR4−/−platelet with or without 5 μg ml−1anti-HMGB1 for 24 h. The levels of total and free active TGFβ1 in the medium were determined by ELISA (Student’st-test). (e) B16F10 or LLC cells were seeded in Matrigel invasion chambers and treated with WT orTLR4−/−platelets with or without 5 μg ml−1anti-HMGB1 for 24 h (LLC) or 36 h (B16F10). The migrated cells were counted (Student’st-test). (f) Mice were injected with B16F10 cells i.v. and treated with anti-HMGB1 as described in ‘Methods’. Fourteen days later, the mice were killed and the lung tumour load was evaluated. Representative picture is shown (Mann–WhitneyU-test;n=5 per group). *P<0.05; **P<0.01. Data are representative of at least three independent experiments. Error bars represent s.e.m. Figure 7: HMGB1 plays a crucial role in platelet–tumour cell interaction. ( a ) The levels of HMGB1 in the plasma of tumour-bearing mice were detected by ELISA. (Student’s t -test; n =5 per group). ( b ) The levels of HMGB1 in the plasma of mice with spontaneous LLC metastases were detected by ELISA. (Student’s t -test; n =5 per group). ( c ) Platelet adhesion to B16F10 or LLC cells with or without 5 μg ml − 1 anti-HMGB1 was quantified based on the fluorescence detection of CFSE-labelled platelets as described in ‘Methods’ (Student’s t -test). ( d ) B16F10 or LLC cells were co-cultured with WT or TLR4 −/− platelet with or without 5 μg ml − 1 anti-HMGB1 for 24 h. The levels of total and free active TGFβ1 in the medium were determined by ELISA (Student’s t -test). ( e ) B16F10 or LLC cells were seeded in Matrigel invasion chambers and treated with WT or TLR4 −/− platelets with or without 5 μg ml − 1 anti-HMGB1 for 24 h (LLC) or 36 h (B16F10). The migrated cells were counted (Student’s t -test). ( f ) Mice were injected with B16F10 cells i.v. and treated with anti-HMGB1 as described in ‘Methods’. Fourteen days later, the mice were killed and the lung tumour load was evaluated. Representative picture is shown (Mann–Whitney U -test; n =5 per group). * P <0.05; ** P <0.01. Data are representative of at least three independent experiments. Error bars represent s.e.m. Full size image In sum, these data indicate that HMGB1 is one of the key factors released by tumour cells, signalling through TLR4 to activate platelets and thus promote tumour metastasis. Most studies linking TLR4 and its ligand LPS with metastasis [16] , [17] were focused on tumour cell TLR4. In the present study, we demonstrate that host TLR4 also plays a key role in supporting metastasis. When tumour cells were administered to TLR4 -deficient mice, lung colonization of the i.v.-injected cells and spontaneous metastasis from subcutaneous primary tumour were markedly curtailed. However, host TLR4 deficiency did not affect the primary (subcutaneous) or secondary (pulmonary) tumour growth. Although it is reported that LPS-induced growth and metastasis of experimental lung metastases is associated with increased angiogenesis, vascular permeability and tumour cell invasion/migration [16] , our data suggest that host TLR4 did not affect the angiogenesis in tumours, at least in our model. It seemed more likely to be that the explanation for decreased tumour dissemination in TLR4 −/− mice lies in an altered tumour–host interaction. We thus reasoned that fewer metastatic foci observed in TLR4 −/− mice were due to diminished B16F10 engraftment into the lung. At early time points, fewer B16F10 cells were retained in the lungs of TLR4 −/− mice. LLC cells also showed a trend towards diminished 6-h lung retention in TLR4 −/− mice. Therefore, impaired metastasis could result from decreased tumour cell survival in the circulation and/or engraftment in the target sites. TLR4 activation on tumour cells facilitates escape from immune surveillance [26] and promotes EMT [17] . In accordance, LPS treatment in TLR4 -null mice led to increased metastasis, although the amplitude was smaller than in WT mice. On the contrary, blockage of TLR4 using TAK-242 inhibited tumour metastasis in WT mice rather than in TLR4 −/− mice. These data definitely demonstrate that in our experiment model, activation of TLR4 expressed on host cells but not tumour cells promoted metastasis. Metastasis is not only a function of tumour cells but is also a process involving cooperative interactions with host cells, in particular platelets and leukocytes. These host cells alter the behaviour of the tumour cells and of endothelial cells lining the vasculature, and assist in tumour cell arrest and extravasation at sites of metastasis, and subsequently in the establishment of tumour foci in the early metastatic niche [4] . BMT experiment showed that TLR4 expressed on haematopoietic-derived cells is responsible for the metastatic promotion. TLR4 is widely expressed on haematopoietic-derived cells, including T cells, NK cells, macrophages, dendritic cells, platelets and so on [13] , all of which are involved in tumour metastasis. However, flow cytometry showed the proportions of NK, T, NKT and MDSC cells in the spleen, blood and metastatic foci were of no significant difference between tumour-bearing WT and TLR4 −/− mice. Blood tests showed TLR4 −/− mice had lower amount of platelets, which is in accordance with previous reports [19] , [29] . Importantly, compared with tumour-bearing WT mice the platelets were less activated in TLR4 −/− mice, and accordingly the level of TGFβ1, a platelet-derived cytokine, was also decreased in tumour-bearing TLR4 −/− mice. Considering these findings and the important roles of platelets in tumour metastasis [5] , we speculated that TLR4 on platelets may be of great importance in tumour metastasis. Indeed, a platelet pretreatment primed tumour cells for metastasis via TLR4-dependent manner. However, we also noticed that the platelet counts were slightly lower in TLR4 deficiency mice (~75% of the WT mice counts). Given a recent report showing that a substantial reduction of the platelet numbers is required to negatively have an impact on metastasis (≥85%) [6] , it is quite possible that TLR4 deficiency affected metastasis due to defects of a platelet function rather than platelet number. To directly verify this hypothesis, we determined the effects of widely used anti-platelet agents Aspirin and Clopidogrel on tumour metastasis. As expected, these two platelet-activation inhibitors reduced experimental metastasis only in WT mice. Interestingly, the size distribution of metastasis foci formed in WT mice treated with or without anti-platelet agents was of no significant difference, indicating that anti-platelet treatment had little direct effects on tumour cell growth and/or apoptosis. Although it is reported that high dose of aspirin [48] (100 mg kg − 1 per day) can reduce tumour burden and metastasis by direct tumour cell apoptosis and inhibition of angiogenesis, the low dose of aspirin used in our system (10 mg kg − 1 per day) is unlikely to cause such effects [43] . These data suggest that TLR4 deficiency may impair platelet activation during tumour metastasis. The platelet–tumour cell interaction are important for metastasis [49] . These interactions include (a) the activation of platelets by tumour cells and adhesion of platelets to tumour cells; (b) the secretion of cytokines, chemokines and other factors that support metastasis from platelets activated by tumour cells; and (c) the presentation of immunoregulatory molecules on the platelet surface. Thus, we determined whether TLR4 was involved in platelet–tumour cell interaction. Based on a CSFE-labelled platelet method and enzyme-linked immunosorbent assay (ELISA), we did find that TLR4 deficit impaired platelet–tumour cell interaction both in vitro and in vivo , and TGFβ1 release from platelets. Moreover, TLR4 deficiency also attenuated the promoting effects of platelets on tumour migration and invasion both in vitro and in vivo . These data demonstrate that TLR4 on platelets are involved in platelet–tumour cell interaction. An obvious question is how TLR4 affects platelet–tumour cell interaction. The interaction of exogenous LPS (a pathogen-associated molecular pattern) and TLR4 was shown to play an important role in tumour metastasis under apparent endotoxemia [16] . Thus, we speculated that endogenous ligands of TLR4 were the reason for TLR4 activation and subsequently affected platelet–tumour cell interaction. Endogenous ligands including HMGB1, HSP70, Biglycan and HAS1-3 released from damaged or stressed tissues can also signal through TLRs [13] . In the initial hours of metastasis, most tumour cells in the circulation were destroyed by shear stress or immune cells [4] , and the alarmin protein HMGB1 can be released by dying tumour cells and activate dendritic cells [15] . In the present study, we found that HMGB1 was presented in the plasma of tumour-bearing mice. Importantly, HMGB1 was present in the tumour cell-derived microvesicles, indicative of active secretion from tumour cells. By using anti-HMGB1 antibody, we found that neutralization of HMGB1 abolished the effects of WT platelets but not TLR4 −/− platelets on tumour cells. However, the roles of other endogenous ligands and the synergetic mechanisms by which LPS and endogenous ligands may contribute to activation of TLR4 pathway in tumour metastasis need further investigation. In conclusion, our data impose the importance of the TLR4 on platelets in the tumour metastasis. Our data show that interaction between tumour cell-derived HMGB1and TLR4 on platelets leads to platelet activation, enhances platelet–tumour cell interactions and thus promotes tumour metastasis. As depletion of platelets or anti-platelet activation using antibodies or pharmacological methods may have side effects such as haemorrhage, inhibition of TLR4 activation by inhibiting HMGB1 released from tumour cells may be an optimal approach to prevent and treat tumour metastasis. Animals Male WT (C57BL/10SnJ) and TLR4 -deficient ( TLR4 −/− ; C57BL/10ScNJ) mice were obtained from the Model Animal Research Center of Nanjing University, Nan Jing, and maintained at an animal facility under pathogen-free conditions. C57BL/6 mice were purchased from China Academy of Science. The mice used in all experiments were male, 6–8 weeks old and of 22–26 g weight. All animals received humane care according to the criteria outlined in the ‘Guide for the Care and Use of Laboratory Animals’ and the animal experiments protocols were approved by the Institutional Animal Care and Use Committee of the Second Military Medical University. Cell culture Murine cell lines B16F10 and LLC were obtained from Shanghai Cell Bank (Shanghai, China) and cultured in RPMI 1640 or DMEM, respectively, with 10% fetal bovine serum (FBS) within a humidified incubator containing 5% CO 2 at 37 °C. In vivo tumour experiments For primary tumour growth, 2 × 10 5 B16F10 or LLC cells were injected subcutaneously. The longest (length) and shortest (width) diameters of the tumours were measured using a sliding caliper every 2 days and the volumes were calculated (length × width 2 × 0.52). For experimental lung metastasis, B16F10 and LLC cells were trypsinized, resuspended in PBS and then 5 × 10 5 cells or indicated number of cells (in 0.1 ml PBS) were injected via the lateral tail vein using a 27-gauge needle. Mice were killed 14–15 days (B16F10) or 21 days (LLC) after injection and the lungs were isolated and fixed in 10% neutral-buffered formalin. Surface metastatic foci in the lung were counted under a dissecting microscope and the nodule size was measured. For spontaneous metastasis, WT and TLR4 −/− mice were injected with 5 × 10 5 LLC cells (a kind gift from Professor Wei Zhang, East China Normal University) subcutaneously. The primary tumour was resected 12 days later. Four weeks after tumour resection, the mice were killed and the surface metastatic nodules on the lungs were counted. In some experiments, B16F10 and LLC cells were labelled for 15 min at 37 °C with 10 μg ml − 1 CFSE (Life Technologies, Canada) in serum-free medium, washed twice and 1 × 10 6 cells were injected i.v. slowly (~2 min per injection to prevent clumping). After 6 h, mice were killed and surface metastatic loci in the lung were counted using Olympus SZX12 fluorescent stereomicroscope (Olympus, Japan). In some experiments, mice were administered with 2 mg kg − 1 LPS from Escherichia coli O55:B5 (Sigma-Aldrich, St Louis, MO) i.p. 6 h before B16F10 cell injection. To block TLR4, mice were injected with 1 mg kg − 1 TAK-242 (Chembest, China) i.p. 1 h before tumour cell infusion. Engraftment of tumour cells in the lung CFSE-labelled B16F10 cells (5 × 10 5 per mouse) were i.v. injected into WT or TLR4 − / − mice. The mice were i.v. injected with DyLight 594- Lycopersicon esculentum (Tomato) lectin (100 μl per mouse) 6 h later. After 10 min, lung tissues of mice were cryosectioned (10 μm) for fluorescence imaging to visualize the vasculature (red) and engrafted tumour cells (green). The tumour cells overlapping with vasculature were considered as circulating cells. Otherwise, the cells away from lectin-positive vasculature were considered as extravasated ones. Five fields (× 200) from each mouse were randomly chosen for fluorescence imaging, and three mice for each group. Bone marrow transplantation WT mice were lethally irradiated with 9.0 Gy using a cobalt-source γ-irradiator. Irradiated recipient mice were i.v. injected with ~1 × 10 7 bone marrow cells in 200 μl of PBS. To demonstrate the success of BMT in mice, the blood and bone marrow of the chimeric mice were collected and genomic DNA was extracted. The presence of the Tlr4 gene was measured by means of quantitative PCR [14] . The Tlr4 primers were: forward: 5′- GCAACTTGGACCTG -3′; reverse: 5′- ATCTGTGAGCGTGTAT -3′. The protocol for quantitative PCR was as follows: 95 °C for 5 min; 95 °C for 30 s, 56 °C for 30 s and 72 °C for 35 s, (30cycles), and 72 °C for 5 min. Anti-platelet drug treatment Mice injected with 5 × 10 5 B16F10 were assigned to receive Aspirin (Asp), Clopidogrel (Clo), Asp/ Clo, or diluents (Vehicle). Asp (Sigma-Aldrich) was administered (alone or in combination with Clo) in the drinking water at the concentration of 100 mg l − 1 . This dose was chosen based on the actual water intake of C57BL/6 mice (~3 ml per dayfor a 30 g mouse), such that the cumulative daily dose of Asp was ~10 mg kg − 1 per day. The drinking water, with or without the addition of aspirin, was replaced every other day. Clo hydrogen sulfate (Sanofi Pharma Bristol, France) was dissolved in 0.003% HCl and administered (alone or in combination with Asp) through drinking water containing 20 μg ml − 1 . The cumulative daily dose of Clo was ~2 mg kg − 1 of body weight. Vehicle-treated mice received identical drinking water supplemented with identical amounts of the Clo-related diluent (0.003% HCl). Platelet isolation from mouse blood Whole blood was drawn from anaesthetized mice via the retroorbital plexus and collected in citric acid–citrate–dextrose solution (85 mM trisodium citrate, 67 mM citric acid, 111.5 mM glucose, pH 4.5; 1:6 blood vol/vol). The blood was centrifuged at 180 g at room temperature for 10 min to obtain platelet-rich plasma (PRP), which was centrifuged at 1,800 g for 5 min to obtain platelet pellet. The platelets were washed twice in CGS buffer (13 mM trisodium citrated, 30 mM dextrose and 120 mM NaCl, pH 7.0) in the presence of 1 μg ml − 1 PGE 1 (Sigma-Aldrich). Washed platelets were resuspened at a concentration of 1 × 10 9 ml − 1 in Tyrode’s buffer (138 mM NaCl, 2.9 mM KCl, 12 mM NaHCO 3 , 0.36 mM NaH 2 PO 4 , 5.5 mM glucose, 1 mM CaCl 2 and 1 mM MgCl 2 , pH 7.4) containing 0.2% BSA. Treatment of tumour cells with platelets for in vitro assay B16F10 or LLC cells were seeded in the corresponding medium with 10% FBS and incubated overnight. Immediately before treatment, the medium was changed for fresh medium. A total of 1.5 × 10 8 platelets per ml were added. Flow cytometry For detecting the P-selectin expression on platelets, PRP were isolated from tumour-bearing mouse and incubated with fluorescein isothiocyanate–P-selectin (1 μg ml − 1 ; BD Biosciences, Franklin Lakes, NJ) at room temperature for 15 min. Next, the PRPs were centrifuged and washed. The P-selectin expression was detected using Moflo-XDP system (Beckman-Coulter). The isolation of splenocytes and flow cytometry for detecting the splenic cells was performed as described previously [50] . Briefly, after the mouse was killed by CO 2 inhalation, the spleen was surgically removed, kept on ice in sterile RPMI1640 supplemented with 1% FBS and pressed through a cell strainer (70 μm Nylon). Next, homogenized cell suspension was washed twice with RPMI1640 by centrifugation at 400 g for 10 min. After the red blood cells were lysed using ammonium chloride lysing reagent (0.15 M NH 4 Cl, 1 mM KHCO 3 , 0.1 mM EDTA), the cell pellet were resuspended in RPMI1640 for antibody labelling and flow cytometry. The NK cells were defined as NK1.1 + CD3 − splenocytes, the T cells were defined as NK1.1 − CD3 + splenocytes, the NKT cells were defined as NK1.1 + CD3 + splenocytes and MDSC cells were defined as CD11b + Gr-1 + splenocytes. Monoclonal antibodies to mouse CD3 (PE), NK1.1 (fluorescein isothiocyanate), CD11b (PE) and Gr-1 (APC) were all from Biolegend (San Diego, CA), and the dilution of the antibodies was 1:100. The peripheral blood mononuclear cells were isolated using lymphocyte separation liquid. To isolate the mononuclear cells in the tumour-bearing lungs, mice were anaesthetized and the lung was perfused through pulmonary artery for 5 min. Next, the lung was isolated and pressed through a 200-gauge stainless steel mesh. After one washing, the cells were resuspended in 40% Percoll (Invitrogen) solution and centrifuged at 2,400 r.p.m. for 30 min at room temperature. The cell pellet were resuspended and incubated with indicated antibodies. Platelet adhesion assay The platelet adhesion assay was performed as previously described [51] . In brief, B16F10 or LLC cells were seeded in a 96-well plate (black with clear bottom; Corning, NY) at a concentration of 5 × 10 4 per 100 μl and grown until confluent. Washed platelets (1.5 × 10 8 per ml) preloaded with CFSE (5 μg ml −1 ) were allowed to adhere to the cells for 45 min at 37 °C. The total fluorescence (485/535 nm) per well was measured using multilabel counter (BioTek, Winooski, VT) plate reader. The plate was washed three times, 100 μl of medium was added to each well of the plate and the remaining fluorescence was read. Percentage platelet adhesion was calculated as (remaining fluorescence−blank)/(total fluorescence−blank) × 100. Platelet infusion Washed platelets (1 × 10 9 in 0.2 ml PBS) were injected into mice via the lateral tail vein immediately after 5 × 10 5 B16F10 cells injection via the other lateral tail vein. The platelets were infused every 5 days. Tumour cells pretreated with platelets for in vivo assay B16F10 cells were seeded in a 10-cm plate. After growth to 50–60% confluence, platelets (1.5 × 10 8 ml − 1 ) were added into the plate and cultured for 40 h, and then washed, harvested and resuspended in PBS at a concentration of 5 × 10 6 ml − 1 . Cell suspension (0.1 ml) was injected into mice i.v. Platelet adhesion to tumour cell assay by microscopy To determine platelets adhering to tumour cells in vitro , tumour cells were seeded in 3.5 mm dish and grown until confluent. Platelets (1.5 × 10 8 per ml) stained with CFSE (5 μg ml −1 ) were added into tumour cells and allowed to adhere to the cells for 45 min at 37 °C. Next, the cells were washed three times with PBS and fixed with 4% formaldehyde. The adherent platelets around tumour cells were photographed with a Leica Confocal microscope. To determine platelets adhering to tumour cell in vivo , WT mice were injected with 100 μg anti-CD41 antibody i.v. (Clone MWReg30; Biolegend) to induce thrombocytopenia. B16F10 cells were stained with PKH26 (Sigma-Aldrich) following the manufacturer’s instruction. Three hours after anti-CD41antibody infusion, 5 × 10 5 PKH26-B16F10 were injected into mice through the lateral tail vein, and immediately 1 × 10 9 CFSE-labelled platelets were injected into mice through the other lateral tail vain. Six hours later, the lungs were isolated, embedded in O.C.T compound (Tissue-Tek) and frozen in liquid nitrogen. The 10-μm-lung sections were determined using a Leica Confocal microscope (Leica Microsystems) and the number of B16F10 cells (red) surrounded with platelets (green) were counted. Enzyme-linked immunosorbent assay TGFβ1 levels were detected in the platelet-treated tumour cell medium (24 h) or platelet-poor plasma by direct assay (active TGFβ1) using the free active TGFβ1 detection kit (Biolegend), or following acid treatment to activate latent TGFβ1 (total TGFβ1) with the TGFβ1 immunoassay kit (Lianke Bio, China) according to the manufacturer’s instruction. The levels of HMGB1 in the plasma of tumour-bearing mice were determined by ELISA (Chondrex, Redmond, WA) according to the manufacturer’s instruction. Soluble P-selectin levels were detected in the platelet-poor plasma by ELISA using a mouse soluble P-selectin ELISA kit (R&D). TXA2 levels were measured by enzyme immunoassay (Cayman Chemical, USA) for its stable breakdown product TXB2. Immunoblotting Immunoblotting analysis was performed as described previously [14] . The primary antibody anti-HMGB1 (1:1,000) were purchased from Abcam, UK; the anti-β-actin antibody (1:200) were obtained from Santa Cruz Biotechnology, Inc.; and the anti-TSG101 antibody (1:1,000) were obtained from ABclonal Biotech Co., Ltd. Migration and invasion assay Tumour cell migration assay were performed using a transwell plate (Corning Costar, NY) with 8 μm insert. Tumour cells (1 × 10 5 ) in 0.1 ml serum-free medium were seeded in the insert (upper chamber) and treated with 1.5 × 10 8 per ml platelets. The lower chamber was added with 0.6 ml medium containing 10% FBS. After 24 h, cells remaining in the upper part of the transwell were removed with a cotton swab. Migrated cells were then stained with Crystal Violet 0.5% and the number of cells was counted per high field (× 200) with an Olympus microscope. Invasion assays were performed in 24-well BD Biocoat Matrigel Invasion Chambers (8 μm pore size; BD Biosciences). Cells (2 × 10 5 ) in 0.2 ml serum-free medium were plated in transwell inserts and either left untreated, anti-HMGB1 blocking antibody and/or 1.5 × 10 8 per ml platelets. The lower chambers contained medium with 10% FBS. After 24 h (LLC) or 36 h (B16F10), migrated cells were counted as migration assay. In some experiments, TGFβRI inhibitor SB431542 (Sigma-Aldrich) were added to the cell culture at a concentration of 10 μM. In some experiments, platelets (1.5 × 10 8 per ml) were added in the lower chamber to determine the necessity of direct contact between platelets and tumour cells for tumour cell invasion. Anti-HMGB1 antibody treatment The anti-HMGB1 antibody was described previously [47] . For in vitro assay, cells were treated with 5 μg ml − 1 anti-HMGB1 antibody or non-immune mouse IgG (Sigma-Aldrich; served as control). For in vivo study, mice were administrated with 50 μg anti-HMGB1 antibody or control IgG i.v. immediately after B16F10 cells inoculation, and once a day for the next 3 days. Fourteen days later, the mice were killed and the lung tumour load was evaluated. Isolation of microvesicles and exosomes Microvesicles and exosomes were isolated from cell culture supernatant. FBS used in culture media for exosome isolation was pre-cleared by ultracentrifugation at 100,000 g for 3 h at 4 °C. Tumour cells at 80% of confluency were incubated for 24 h in exosome-depleted FBS medium. Next, the medium was collected and centrifuged at 1,500 g for 10 min to eliminate cellular debris. The supernatant was centrifuged at 20,000 g for 30 min to isolate microvesicles. The rest supernatant was filtered through 0.22 μm filter (Millipore), concentrated using Amicon Ultra-4 (100 kD cutoff) filter units (Millipore) and then centrifuged at 100,000 g for 90 min to isolate exosomes using the Beckman Coulter Max-XP Ultracentrifuge with a TLS-55 Swing-Bucket Rotor. Statistical analysis Normally distributed data were presented as mean±s.e. and analysed by Student’s t -test. Non-normally distributed data were analysed using Mann–Whitney U -test. Statistical significance was assumed when P <0.05. How to cite this article: Yu, L.-X. et al . Platelets promote tumour metastasis via interaction between TLR4 and tumour cell-released high-mobility group box1 protein. Nat. Commun. 5:5256 doi: 10.1038/ncomms6256 (2014).